Early aqueous activity on the ordinary and carbonaceous chondrite parent bodies recorded by fayalite Chronology of aqueous activity on chondrite parent bodies constrains their accretion times and thermal histories. Radiometric 53 Mn– 53 Cr dating has been successfully applied to aqueously formed carbonates in CM carbonaceous chondrites. Owing to the absence of carbonates in ordinary (H, L and LL), and CV and CO carbonaceous chondrites, and the lack of proper standards, there are no reliable ages of aqueous activity on their parent bodies. Here we report the first 53 Mn– 53 Cr ages of aqueously formed fayalite in the L3 chondrite Elephant Moraine 90161 as Myr after calcium–aluminium-rich inclusions (CAIs), the oldest Solar System solids. In addition, measurements using our synthesized fayalite standard show that fayalite in the CV3 chondrite Asuka 881317 and CO3-like chondrite MacAlpine Hills 88107 formed and Myr after CAIs, respectively. Thermal modelling, combined with the inferred conditions (temperature and water/rock ratio) and 53 Mn– 53 Cr ages of aqueous alteration, suggests accretion of the L, CV and CO parent bodies ∼ 1.8−2.5 Myr after CAIs. Most chondritic meteorites (chondrites) experienced aqueous alteration resulting in the formation of a diverse suite of secondary minerals, including phyllosilicates, magnetite (FeFe 2 O 4 ), sulfides, carbonates (calcite (CaCO 3 ), dolomite (CaMg(CO 3 ) 2 ), breunnerite (Mg,Fe,Mn)CO 3 ) and siderite (FeCO 3 )), ferromagnesian olivines ((Fe,Mg) 2 SiO 4 ) and Ca-rich pyroxenes (Ca(Fe,Mg)Si 2 O 6 ; ref. 1 ). Mineralogical observations, isotopic data and thermodynamic analysis suggest that the alteration resulted from interactions between a rock and an aqueous solution in an asteroidal setting [2] . Therefore, dating minerals formed by aqueous alteration provides important constraints on the accretion ages of chondrite parent bodies. The chondrite accretion ages, the conditions of aqueous alteration (temperature and water/rock ratio), and the inferred hydrogen and oxygen isotopic compositions of chondritic water [3] , [4] can potentially be used to constrain chondrite accretion regions and to test the recently proposed Grand Tack dynamical model of the early Solar System evolution [5] . According to this model, the hydrated P-type, D-type and taxonomic C-complex asteroids, which are commonly associated with carbonaceous chondrites [6] , accreted outside Jupiter’s orbit (5–15 AU from the Sun; 1 AU is the distance between the Sun and the Earth), and were scattered and implanted into the main asteroid belt (located between 2 and 4 AU from the Sun) during the migration of Jupiter and Saturn within the first several million years of the Solar System formation. The short-lived radionuclide 53 Mn, which decays to 53 Cr with a half-life of ∼ 3.7 Myr and appears to have been uniformly distributed in the protoplanetary disk [7] , is known to be a useful tool for dating aqueous alteration [1] . As yet, accurate 53 Mn– 53 Cr ages of aqueous alteration are only known for the CM (Mighei-like) carbonaceous chondrites [8] containing aqueously formed Mn-rich, Cr-poor calcite suitable for in situ radiometric 53 Mn– 53 Cr dating with secondary ion mass spectrometry (SIMS). SIMS measurements of manganese-chromium (Mn–Cr) isotope systematics of a mineral require a proper standard to determine a relative sensitivity factor (RSF=( 55 Mn + / 52 Cr + ) SIMS /( 55 Mn/ 52 Cr) mineral ) to correct for the relative sensitivities between 55 Mn + and 52 Cr + ions and to calculate true 55 Mn/ 52 Cr ratios in the mineral. The initial 53 Mn/ 55 Mn ratio, ( 53 Mn/ 55 Mn) 0 , of calcites in CM chondrites has been determined by using an RSF measured on a synthetic Mn- and Cr-doped calcite standard [8] . The inferred initial 53 Mn/ 55 Mn ratios, ranging from ∼ 2.7 × 10 −6 to ∼ 3.4 × 10 −6 , correspond to calcite formation ages of ∼ 4−5 Myr after the formation of calcium–aluminium-rich inclusions (CAIs), the oldest Solar System solids dated [9] . Carbonates, however, are virtually absent in weakly aqueously altered ordinary (H, L and LL) and several carbonaceous chondrite groups, including CV (Vigarano-like) and CO (Ornans-like). Instead, the least metamorphosed meteorites of these groups contain aqueously formed Mn-rich, Cr-poor fayalite (Fa >90 ; Fayalite (Fa) number=atomic Fe/(Fe+Mg) × 100 in olivine) suitable for in situ Mn–Cr isotope dating with SIMS [10] , [11] , [12] . As for carbonates, SIMS measurements of 53 Mn– 53 Cr systematics in fayalite require a proper standard to determine the RSF and calculate 55 Mn/ 52 Cr ratios. Because natural fayalite contains virtually no chromium, it cannot be used as a standard for Mn–Cr isotope measurements; San Carlos olivine (Fa 10 ) was typically used instead [10] , [11] , [12] . However, it has been recently discovered that the RSF in olivine changes as a function of its fayalite content [13] , [14] . Therefore, all previously published 53 Mn– 53 Cr ages of CV and CO chondritic fayalite, acquired with a San Carlos olivine standard [10] , [11] , [12] , need to be corrected. To obtain accurate 53 Mn– 53 Cr ages of fayalite, a Mn- and Cr-doped fayalite (Fa 99 ) standard was synthesized (ref. 14 and Doyle et al. , manuscript in preparation). Here we report on the mineralogy, petrography and oxygen-isotope compositions of the fayalite-bearing assemblages and 53 Mn– 53 Cr ages of fayalite in type 3 L, LL, CO and CV chondrites. Our data confirm the origin of fayalite during low-temperature aqueous alteration on the L, CV and CO chondrite parent bodies [10] , [11] , [12] , and allow us to constrain the accretion ages and the accretion regions of these bodies. 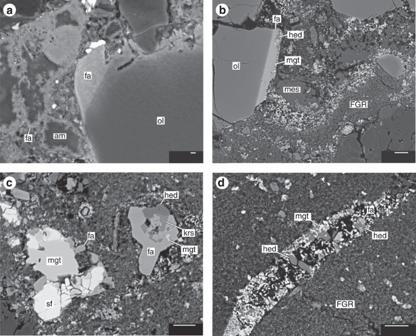Figure 1: Textural occurrences of fayalite-bearing assemblages in ordinary and carbonaceous chondrites. Backscattered electron images of fayalite-bearing assemblages in (a) ordinary and (b−d) carbonaceous chondrites. Shown are (a) two occurrences of fayalite (fa) in the OC EET 90161 (L3.05): fayalite overgrows onto an Mg-rich chondrule olivine (ol) and replaces amorphous (am) material; and (b−d) three occurrences of fayalite–hedenbergite (hed)–magnetite (mgt) assemblages in the CO3-like carbonaceous chondrite MAC 88107. (b) Ferroan porphyritic chondrule (type II) surrounded by a fine-grained rim (FGR). Chondrule mesostasis (mes) is replaced by phyllosilicates and partially leached out. The olivine phenocryst at the boundary with the mesostasis is overgrown by fayalite with inclusions of hedenbergite and magnetite. (c) Fe,Ni-sulfide (sf)–magnetite–fayalite–hedenbergite–kirschsteinite (krs) particles in the hydrated (phyllosilicate-bearing) matrix. (d) Fine-grained rim around magnesian porphyritic chondrule (type I) is crosscut by a vein composed of magnetite, fayalite and hedenbergite. Scale bars, 1 μm (a) and 10 μm (b−d). Petrographic evidence for in situ formation of fayalite Nearly pure fayalite (Fa 90−100 ; Supplementary Table 1 ) was found in the aqueously altered ordinary (Semarkona (LL3.00), Elephant Moraine (EET) 90161 (L3.05), Meteorite Hills (MET) 00452 (L/LL3.05), MET 96503 (L3.1–3.2), Ngawi (LL3–6)) and carbonaceous (MacAlpine Hills (MAC) 88107 (CO3-like) and Asuka (A) 881317 (CV3)) chondrites. There are three major textural occurrences of fayalite in these meteorites: (1) fayalite with tiny inclusions of hedenbergite (CaFeSi 2 O 6 ) and magnetite overgrows onto ferromagnesian chondrule olivines (Fa 1−30 ; Fig. 1a,b ). There are sharp compositional boundaries between the fayalite and the chondrule olivines. These observations are consistent with low-temperature formation of the fayalite overgrowths and the lack of subsequent thermal metamorphism above ∼ 300–400 °C that would have resulted in Fe–Mg interdiffusion between the adjacent fayalite and ferromagnesian olivines. (2) In the hydrated chondrite matrices, fayalite associates with hedenbergite, magnetite and Fe,Ni-sulfides, and often forms euhedral crystals that show no evidence for corrosion or replacement by the surrounding phyllosilicates. These observations indicate a local equilibrium between the fayalite and the phyllosilicates ( Fig. 1c ). In addition, in matrices of the ordinary chondrites (OCs) EET 90161, MET 96503 and MET 00452, fayalite replaces amorphous ferromagnesian silicates ( Fig. 1a ). (3) Fine-grained matrix-like rims around magnesian porphyritic chondrules in MAC 88107 and A-881317 are commonly crosscut by veins composed of fayalite, hedenbergite and magnetite ( Fig. 1d ), indicating in situ crystallization of this mineral paragenesis. Figure 1: Textural occurrences of fayalite-bearing assemblages in ordinary and carbonaceous chondrites. Backscattered electron images of fayalite-bearing assemblages in ( a ) ordinary and ( b − d ) carbonaceous chondrites. Shown are ( a ) two occurrences of fayalite (fa) in the OC EET 90161 (L3.05): fayalite overgrows onto an Mg-rich chondrule olivine (ol) and replaces amorphous (am) material; and ( b − d ) three occurrences of fayalite–hedenbergite (hed)–magnetite (mgt) assemblages in the CO3-like carbonaceous chondrite MAC 88107. ( b ) Ferroan porphyritic chondrule (type II) surrounded by a fine-grained rim (FGR). Chondrule mesostasis (mes) is replaced by phyllosilicates and partially leached out. The olivine phenocryst at the boundary with the mesostasis is overgrown by fayalite with inclusions of hedenbergite and magnetite. ( c ) Fe,Ni-sulfide (sf)–magnetite–fayalite–hedenbergite–kirschsteinite (krs) particles in the hydrated (phyllosilicate-bearing) matrix. ( d ) Fine-grained rim around magnesian porphyritic chondrule (type I) is crosscut by a vein composed of magnetite, fayalite and hedenbergite. Scale bars, 1 μm ( a ) and 10 μm ( b − d ). Full size image Oxygen isotopic compositions Oxygen isotopic compositions of fayalite, magnetite, chondrule olivines and the bulk compositions of type 3 ordinary, CV and CO chondrites are plotted on a three-isotope oxygen diagram, δ 17 O versus δ 18 O ( Fig. 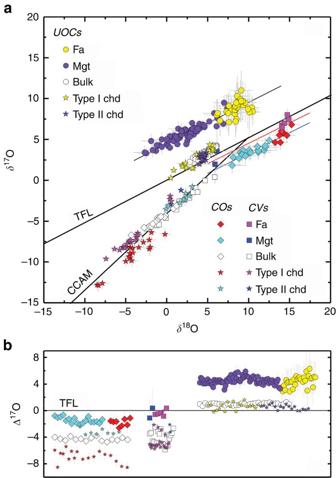Figure 2: Oxygen isotopic compositions of fayalite-bearing assemblages and chondrule olivines. (a) Three-isotope oxygen diagram (where δ17,18O=[(17,18O/16Osample)/(17,18O/16OSMOW) −1] × 1,000 and SMOW is standard mean ocean water) showing the compositions of fayalite (Fa), magnetite (Mgt), chondrule (chd) olivine fragments, and bulk compositions for EET 90161 and other unequilibrated OCs (UOCs), A-881317 (CV3), MAC 88107 (CO3-like) and other CO and CV carbonaceous chondrites. The terrestrial fractionation line (TFL) and CCAM line are shown for reference. (b) Δ17O values of fayalite, magnetite, chondrule fragments and bulk compositions of UOCs, CO and CV chondrites. The data are plotted arbitrarily on thexaxis to show individual compositions. The difference in Δ17O observed between chondrule olivines and the secondary minerals (fayalite and magnetite) indicate that they are in isotopic disequilibrium, which is consistent with the low-temperature formation of fayalite and magnetite. Uncertainties shown are 2σ. Fayalite and magnetite data are from EET 90161, Semarkona (LL3.00), MET 00452 (L/LL3.05) and Ngawi (L3–6 breccia) (Supplementary Table 2). Bulk meteorite and chondrule compositions from refs15,16,17,18,19. 2a and Supplementary Table 2 ). In Fig. 2b , the same data are plotted as deviation from the terrestrial fractionation line, Δ 17 O=δ 17 O − 0.52 × δ 18 O. Figure 2: Oxygen isotopic compositions of fayalite-bearing assemblages and chondrule olivines. ( a ) Three-isotope oxygen diagram (where δ 17,18 O=[( 17,18 O/ 16 O sample )/( 17,18 O/ 16 O SMOW ) −1] × 1,000 and SMOW is standard mean ocean water) showing the compositions of fayalite (Fa), magnetite (Mgt), chondrule (chd) olivine fragments, and bulk compositions for EET 90161 and other unequilibrated OCs (UOCs), A-881317 (CV3), MAC 88107 (CO3-like) and other CO and CV carbonaceous chondrites. The terrestrial fractionation line (TFL) and CCAM line are shown for reference. ( b ) Δ 17 O values of fayalite, magnetite, chondrule fragments and bulk compositions of UOCs, CO and CV chondrites. The data are plotted arbitrarily on the x axis to show individual compositions. The difference in Δ 17 O observed between chondrule olivines and the secondary minerals (fayalite and magnetite) indicate that they are in isotopic disequilibrium, which is consistent with the low-temperature formation of fayalite and magnetite. Uncertainties shown are 2 σ . Fayalite and magnetite data are from EET 90161, Semarkona (LL3.00), MET 00452 (L/LL3.05) and Ngawi (L3–6 breccia) ( Supplementary Table 2 ). Bulk meteorite and chondrule compositions from refs 15 , 16 , 17 , 18 , 19 . Full size image Oxygen isotopic compositions of fayalite and magnetite in type 3 OCs plot along a mass-dependent fractionation line with a slope of ∼ 0.5 ( Fig. 2a ). The compositions of fayalite and magnetite, having an average Δ 17 O value of +4.8±1.7‰ (2 s.d. ), are significantly different from those of chondrule olivines [15] and bulk OCs [16] , which both have Δ 17 O values of ∼ +1‰ ( Fig. 2b ). Oxygen isotopic compositions of fayalite and magnetite in A-881317 (CV3) plot along a mass-dependent fractionation line with a slope of ∼ 0.5 ( Fig. 2a ) and have an average Δ 17 O value of −0.4±0.9‰ ( Fig. 2b ), consistent with the previously published data for fayalite and magnetite from the Kaba and Mokoia CV3 chondrites [17] . The bulk oxygen isotopic compositions of CV chondrites [18] and CV chondrule olivines [19] plot along the carbonaceous chondrite anhydrous mineral (CCAM) line with a slope of ∼ 1 ( Fig. 2a ) and show a range of Δ 17 O values from −6 to −2‰ ( Fig. 2b ). Oxygen isotopic compositions of fayalite and magnetite in MAC 88107 (CO3-like) plot along a mass-dependent fractionation line with a slope of ∼ 0.5 ( Fig. 2a ) and have an average Δ 17 O value of −1.6±0.9‰ ( Fig. 2b ), whereas chondrule olivines plot along the CCAM line and show a range of Δ 17 O values from −9 to −2‰ ( Fig. 2b ). The bulk oxygen isotopic composition of MAC 88107 also plots along the CCAM line and has a Δ 17 O value of −4.8‰ (ref. 18 ). 53 Mn– 53 Cr ages of fayalite formation To obtain an olivine standard suitable for SIMS measurements of Mn–Cr isotope systematics of chondritic fayalite, we synthesized a suite of ferromagnesian olivines ranging from Fa 31 to Fa 99 (ref. 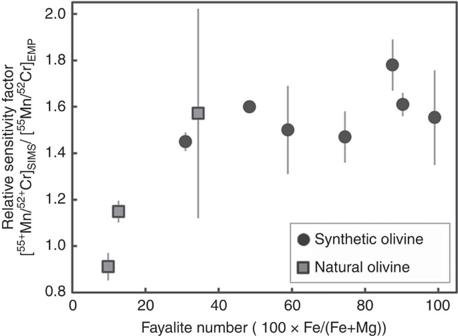Figure 3: Mn–Cr RSF in ferromagnesian olivines. Mn–Cr RSF, determined with the UH Cameca ims-1280 using a primary beam∼5 μm in diameter, as a function of fayalite number. The RSFs reported for samples Fa12–90are an average of 2–7 analyses. Four to five analyses were collected daily from either Fa99or Fa10, and the RSFs reported are an average of 18 and 20 analyses, respectively. The RSFs for Fa10and Fa99collected during individual sessions are shown in Doyleet al.(manuscript in preparation) and described in theSupplementary Discussion. Uncertainties are 2 s.d., with uncertainty in Fa number smaller than the symbols. 14 ; see Methods section and Supplementary Table 3 ). Our Mn–Cr isotope measurements of the synthesized olivine grains with the University of Hawai‘i (UH) ims-1280 SIMS revealed that the RSF strongly depends on the fayalite content in olivine [14] . In olivine with Fa 10–30 , the RSF increases from ∼ 0.9 to ∼ 1.5 as a function of fayalite content; in more ferroan olivines (Fa >30 ), the RSF is nearly constant, ∼ 1.6 ( Fig. 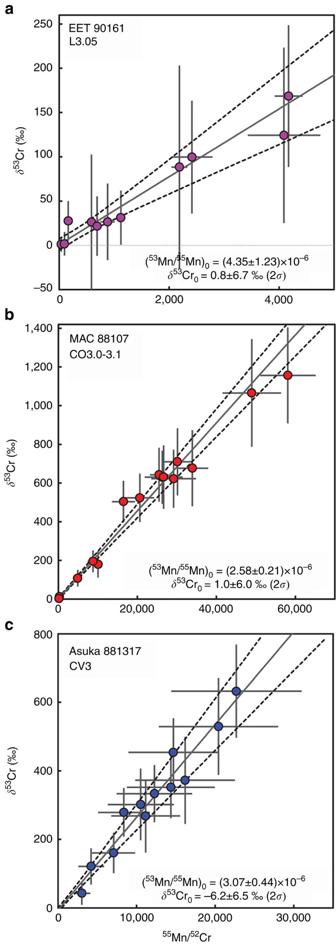Figure 4: Mn–Cr evolutionary diagrams of fayalite in ordinary and carbonaceous chondrites. Mn–Cr evolutionary diagrams of fayalite in (a) EET 90161, (b) MAC 88107 and (c) A-881317. δ53Cr=[(53Cr/52Cr)fayalite/(53Cr/52Cr)terrestrial)-1] × 1,000, where (53Cr/52Cr)terrestrial=0.113459. Excesses of53Cr in the EET 90161, MAC 88107 and A-881317 fayalites are well correlated with55Mn/52Cr, indicative ofin situdecay of53Mn to53Cr. The initial (53Mn/55Mn)0and53Cr/52Cr ratios (δ53Cr0) are indicated in the diagrams. Uncertainties shown are 2σ. 3 and Supplementary Table 4 ). The observed differences in RSF values between fayalite (Fa 90–100 ) and San Carlos olivine (Fa 10 ) suggest that all previously reported 53 Mn– 53 Cr dating of fayalite in carbonaceous chondrites [10] , [11] , [12] are in error and yield systematically young ages [14] . Figure 3: Mn–Cr RSF in ferromagnesian olivines. Mn–Cr RSF, determined with the UH Cameca ims-1280 using a primary beam ∼ 5 μm in diameter, as a function of fayalite number. The RSFs reported for samples Fa 12–90 are an average of 2–7 analyses. Four to five analyses were collected daily from either Fa 99 or Fa 10 , and the RSFs reported are an average of 18 and 20 analyses, respectively. The RSFs for Fa 10 and Fa 99 collected during individual sessions are shown in Doyle et al. (manuscript in preparation) and described in the Supplementary Discussion . Uncertainties are 2 s.d., with uncertainty in Fa number smaller than the symbols. Full size image With the matrix-matched standard (Fa 99 ), we measured Mn–Cr isotope systematics of fayalite in EET 90161, A-881317 and MAC 88107 ( Table 1 and Fig. 4 ). The excess of 53 Cr in fayalite from these meteorites correlates with the 55 Mn/ 52 Cr ratio, indicating in situ decay of 53 Mn. The inferred initial 53 Mn/ 55 Mn ratios in fayalite from EET 90161, A-881317 and MAC 88107 are (4.35±1.23) × 10 −6 , (3.07±0.44) × 10 −6 and (2.58±0.21) × 10 −6 , respectively. Table 1 Mn–Cr isotope compositions of fayalite in EET 90161 (L3.05), MAC 88107 (CO3-like) and A-881317 (CV3). Full size table Figure 4: Mn–Cr evolutionary diagrams of fayalite in ordinary and carbonaceous chondrites. Mn–Cr evolutionary diagrams of fayalite in ( a ) EET 90161, ( b ) MAC 88107 and ( c ) A-881317. δ 53 Cr=[( 53 Cr/ 52 Cr) fayalite /( 53 Cr/ 52 Cr) terrestrial )-1] × 1,000, where ( 53 Cr/ 52 Cr) terrestrial =0.113459. Excesses of 53 Cr in the EET 90161, MAC 88107 and A-881317 fayalites are well correlated with 55 Mn/ 52 Cr, indicative of in situ decay of 53 Mn to 53 Cr. The initial ( 53 Mn/ 55 Mn) 0 and 53 Cr/ 52 Cr ratios (δ 53 Cr 0 ) are indicated in the diagrams. Uncertainties shown are 2 σ . Full size image The 53 Mn– 53 Cr chronometer provides a relative chronology, that is, the 53 Mn– 53 Cr age of mineral formation is given relative to a reference material: Δ t mineral—reference =1/ λ 53Mn × ln[( 53 Mn/ 55 Mn) reference /( 53 Mn/ 55 Mn) mineral ], where λ 53Mn is the decay constant of 53 Mn. In cosmochemistry, the commonly used reference material is CV CAIs, which are the oldest Solar System solids, with the U-corrected Pb–Pb absolute age of 4,567.30±0.16 Ma (ref. 9 ) that is considered to represent the age of the Solar System. The initial 53 Mn/ 55 Mn ratio in CV CAIs has, however, not been measured owing to a lack of primary CAI minerals having high Mn/Cr ratios and the post-crystallization disturbance of their Mn–Cr isotope systematics [20] . Instead, the initial 53 Mn/ 55 Mn ratio in CV CAIs can be calculated from the difference in the U-corrected Pb–Pb ages of CAIs and the U-corrected Pb–Pb ages angrites (basaltic meteorites) with the measured initial 53 Mn/ 55 Mn ratio ( Supplementary Methods ). Using the measured ( 53 Mn/ 55 Mn) 0 in the D’Orbigny angrite of (3.24±0.04) × 10 −6 (ref. 21 ), its U-corrected Pb–Pb absolute age of 4,563.4±0.3 Ma (ref. 22 ) and the U-corrected Pb–Pb absolute age of CV CAIs [9] , the estimated ( 53 Mn/ 55 Mn) 0 ratio in the CV CAIs is ∼ 6.8 × 10 −6 . Therefore, the inferred ( 53 Mn/ 55 Mn) 0 in fayalites from EET 90161, A-881317 and MAC 88107 correspond to the formation ages of , and Myr after the CV CAIs, respectively ( Fig. 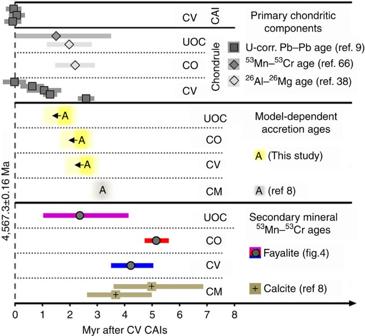Figure 5: Chronology of aqueous alteration and accretion of ordinary and carbonaceous chondrite parent bodies. Chronology of aqueous alteration of unequilibrated OC (UOC: L and LL) and carbonaceous (CO, CV and CM) chondrite parent bodies. Relative ages of fayalite in UOC, CO and CV chondrites, and calcites in CM chondrites8are anchored to the D’Orbigny angrite and shown relative to the age of CV CAIs9(Methods section). Also shown are the model accretion ages of UOC, CO and CV (this study), and CM (8) chondrites, and U-corrected Pb–Pb (9),53Mn–53Cr (ref.66) and26Al–26Mg (ref.38) ages of chondrules in CV, UOC and CO chondrites, relative to the CV CAIs9. 5 and Supplementary Table 5 ). Figure 5: Chronology of aqueous alteration and accretion of ordinary and carbonaceous chondrite parent bodies. Chronology of aqueous alteration of unequilibrated OC (UOC: L and LL) and carbonaceous (CO, CV and CM) chondrite parent bodies. Relative ages of fayalite in UOC, CO and CV chondrites, and calcites in CM chondrites [8] are anchored to the D’Orbigny angrite and shown relative to the age of CV CAIs [9] (Methods section). Also shown are the model accretion ages of UOC, CO and CV (this study), and CM ( [8] ) chondrites, and U-corrected Pb–Pb ( [9] ), 53 Mn– 53 Cr (ref. 66 ) and 26 Al– 26 Mg (ref. 38 ) ages of chondrules in CV, UOC and CO chondrites, relative to the CV CAIs [9] . Full size image Thermal modelling of L, CO and CV chondrite parent bodies Mineral thermometry suggests that L, CV and CO chondrite parent bodies reached peak metamorphic temperatures of ∼ 950, ∼ 600 and ∼ 600 °C, respectively [23] . Thermal evolution of the L-, CV- and CO-like bodies with different radii heated only by decay of the short-lived radionuclide 26 Al, having a half-life of ∼ 0.7 Myr, is modelled with reference to the peak metamorphic temperatures and the ages of fayalite formation in the L, CV and CO chondrites (see Methods section). Our calculations indicate that L chondrite-like bodies with radii of 20−40 km need to accrete within ∼ 1.6–1.8 Myr after CV CAIs, respectively, in order to reach a peak metamorphic temperature of 950 °C ( Fig. 6a ). The CV and CO chondrite-like bodies with radii of 20–50 km need to accrete within ∼ 2.4–2.6 Myr and ∼ 2.1–2.4 Myr after CV CAIs, respectively, to reach a peak metamorphic temperature of 600 °C ( Fig. 6b ). 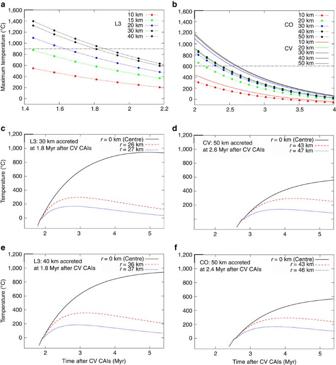Figure 6: Thermal evolution of ordinary and carbonaceous chondrite parent bodies as a function of accretion time and radius. (a,b) Maximum temperature as a function of time after CV CAIs modelled for L, CV and CO chondrite-like parent bodies ranging from 10 to 50 km in radius. (c−f) Temperature evolution diagrams at different depths shown for (c,e) L chondrite-like parent bodies 30 and 40 km in radius; (d) a 50-km radii CV-like parent body; and (f) a 50 km radii CO chondrite-like parent body. The CO chondrites have lower bulk aluminium contents than the CV chondrites ( Supplementary Table 6 ). As a result, the CO chondrite parent body heated by decay of 26 Al must have accreted earlier than the CV chondrite parent body in order to reach the same peak metamorphic temperature. We note that owing to the balance between the heat generated by decay of 26 Al and heat lost through radiation, the maximum temperature reached by a body larger than 30 km in radius largely depends on its accretion time and not its size ( Fig. 6a,b ). Figure 6: Thermal evolution of ordinary and carbonaceous chondrite parent bodies as a function of accretion time and radius. ( a , b ) Maximum temperature as a function of time after CV CAIs modelled for L, CV and CO chondrite-like parent bodies ranging from 10 to 50 km in radius. ( c − f ) Temperature evolution diagrams at different depths shown for ( c , e ) L chondrite-like parent bodies 30 and 40 km in radius; ( d ) a 50-km radii CV-like parent body; and ( f ) a 50 km radii CO chondrite-like parent body. Full size image Temperature evolution at different depths of the L, CV and CO chondrite-like bodies with different sizes and accretion ages are shown in Fig. 6c–f . Regions ∼ 26.5 and ∼ 36.5 km from the centre of L chondrite-like bodies with radii of 30 and 40 km, respectively, would have conditions (100−200 °C) suitable for the formation of fayalite ( Fig. 6c,e ). In a body 30 km in radius, the fayalite-forming region would not have been heated above 300 °C, and would have avoided Fe–Mg diffusion between fayalite and ferromagnesian olivines, consistent with our observations of fayalites in EET 90161. In a body 40 km in radius, the fayalite-forming region would have reached up to 350 °C ∼ 0.5 Myr after fayalite formation, which would have resulted in some Fe–Mg interdiffusion in fayalite. The CV and CO chondrite-like bodies, each with a 50-km radius, have regions ∼ 43−47 km from the centre of the bodies, which experienced metamorphic temperatures in the range of 100−300 °C ( Fig. 6d,f ). These calculations indicate that secondary fayalite is likely to have formed and survived only near the peripheral parts of the L, CV and CO chondrite parent bodies. The oxygen-isotope systematics of fayalite and magnetite in type 3 ordinary and carbonaceous chondrites indicate that these minerals are in isotopic disequilibrium with the chondrule olivines, precluding a high-temperature origin of fayalite and magnetite during chondrule formation [24] . Instead, the large differences in δ 18 O values between the coexisting fayalite and magnetite (up to 10‰ in A-881317 and up to 8‰ in MAC 88107) are consistent with a low-temperature origin of these minerals in equilibrium with an aqueous solution [25] , [26] . The mineralogy, petrography and oxygen isotopic compositions, therefore, support the formation of fayalite-bearing assemblages in type 3 ordinary, CO and CV chondrites during fluid–rock interactions on their respective parent bodies [1] , [10] , [11] , [12] . Thermodynamic analysis of the gas–solution–rock system [27] , [28] shows that nearly pure fayalite (Fa >90 ) is stable at low temperatures ( ∼ 100−200 °C) and low water/rock mass ratios ( ∼ 0.1−0.2), and, therefore, these conditions are inferred for aqueous alteration on the ordinary, CV and CO chondrite parent bodies. These alteration conditions are different from those recorded by the more extensively aqueously altered but less metamorphosed CM and CI (Ivuna-like) carbonaceous chondrites, which have experienced alteration at temperatures of ∼ 20–80 °C (refs 18 , 29 ) and <150–210 °C (refs 18 , 30 ), and water/rock mass ratios of ∼ 0.3−0.6 and >0.8 (ref. 18 ), respectively. The CI and CM chondrites contain abundant phyllosilicates, carbonates and magnetite, but lack fayalite, which is unstable under these alteration conditions [28] . The formation ages of fayalite in L, CO and CV chondrites and the conditions of fayalite stability [28] can be linked to the metamorphic histories and the accretion ages of their parent bodies ( Fig. 6 ). The L chondrites define a metamorphic sequence of petrologic types from 3 to 6, and reached peak metamorphic temperatures of ∼ 950 °C (ref. 23 ). In contrast, the CV and CO chondrites define a narrower range of petrologic types, 3.1 to >3.6 and 3.0 to 3.8, respectively, and reached peak metamorphic temperatures of ∼ 600 °C (refs 23 , 31 , 32 ). As it is not known how well the CV and CO chondrite parent bodies are sampled by the recovered meteorites, the estimated peak metamorphic temperatures provide only a lower limit on the maximum temperatures experienced by these bodies. It is generally accepted that 26 Al was the major heat source responsible for thermal metamorphism and aqueous alteration of early accreted planetesimilas [33] . Assuming 26 Al was homogeneously distributed in the protoplanetary disk with an initial abundance corresponding to the canonical 26 Al/ 27 Al ratio of 5.25 × 10 −5 (refs 34 , 35 , 36 ), we modelled the thermal evolution of several chondrite parent bodies accreting 1.6–4.0 Myr after CV CAIs ( Supplementary Table 6 ). Numerical modelling of an L chondrite-like body with a radius of ∼ 30–40 km ( Fig. 6c,e ) suggests that this body accreted with an initial 26 Al/ 27 Al ratio of ∼ 9 × 10 −6 , corresponding to ∼ 1.8 Myr after CV CAIs. Fayalite could have precipitated ∼ 0.6 Myr later in the outer portion of this body, which may never have experienced temperatures above 300 °C ( Fig. 6c,e ). Similarly, the CV and CO chondrite-like bodies with radii of 50 km ( Fig. 6d,f ) accreted with an 26 Al/ 27 Al ratio of ∼ 4 × 10 −6 corresponding to ∼ 2.5 Myr after CV CAIs. Fayalite could have precipitated ∼ 1.5–2.5 Myr later in the outer portions of these bodies, which may never have experienced temperatures above 300 °C. The modelled accretion age of the CV chondrite parent body is in agreement with the 26 Al– 26 Mg formation age of >2.6 Myr for secondary grossular in the CAIs from the CV3 Allende chondrite [37] . The modelled accretion ages of the L and CO chondrite parent bodies are consistent with the 26 Al– 26 Mg ages of chondrules from the type 3 ordinary and CO chondrites, 1.98±0.82 and 2.19±0.72 Myr after CV CAIs (ref. 38 and references therein), respectively, but require rapid accretion of chondrules after their formation into their parent bodies. The rapid accretion of the chondrite parent bodies after chondrule formation may explain the mineralogical, chemical and isotopic differences between the chondrite groups [39] . The short time interval between the accretion of L, CV and CO chondrite parent bodies and the formation ages of aqueously produced fayalite suggest that the water ices were incorporated into the accreting parent bodies rather than being added later, during regolith gardening. The inferred water/rock mass ratios ( ∼ 0.1–0.2) in ordinary, CO and CV chondrites are much lower than the solar value of 1.2 (ref. 40 ). The estimated low permeability of chondritic meteorites [41] and the lack of variations in bulk chemical compositions between meteorites with different degrees of aqueous alteration [1] , [2] , [42] imply that the alteration occurred in a chemically closed system, with the fluid flow being restricted to 10–100 μm, which is consistent with rare occurrences of short veins in aqueously altered chondrites ( Fig. 1d ). We suggest that the inferred low abundance of water ices in ordinary, CO and CV chondrite parent bodies resulted from their accretion close to the snow line, possibly slightly inside it, where only the relatively large ice-bearing particles could have avoided instantaneous evaporation and survived to be accreted to the parent body [43] . The location of the snow line in the protoplanetary disk is uncertain; it likely did not reside at a single location, but rather migrated with time as the luminosity of the proto-Sun, the mass transport rate through the disk, and the disk opacity all evolved with time. In viscous disks, where mass accretion occurs throughout the disk, energy from internal dissipation can keep the inner disk warm for much of the lifetime of the disk. As mass accretion rates diminished with time, the viscous dissipation would slow, causing the snow line to migrate inwards with time. While specific details vary with the assumed disk structure and viscosity, models [44] , [45] , [46] , [47] suggest that the snow line would be located beyond 5 AU early in disk evolution, but is likely to have been present at 2–3 AU in the 1.8–2.5-Myr-old disk, which corresponds to the accretion ages of ordinary, CV and CO chondrite parent bodies. Thus, this would suggest that the ordinary, CO and CV chondrite parent bodies most likely accreted in the inner part of the Solar System, close to the current position of the main asteroid belt, rather than experiencing large radial excursions that may have occurred during planet migration [5] . This conclusion is inconsistent with the Grand Tack dynamical model of the Solar System evolution that predicts implantation of hydrated carbonaceous chondrite-like planetesimals, formed beyond Jupiter, into the main asteroid belt [5] , [48] . Synthesis experiments To measure the Mn–Cr RSF in fayalite, ferromagnesian olivines covering a wide compositional range (Fa 31–99 ) were synthesized, as described by Doyle et al. (manuscript in preparation). The methodology is summarized as follows: pre-dried Fe 2 O 3 , MgO, SiO 2 , MnCO 3 , Cr 2 O 3 and NiO were mixed in stoichiometric proportions and ground by hand under ethanol. The respective powders were made into a slurry with a polyvinyl alcohol solution and attached to platinum loops. The loops were suspended from a platinum chandelier within a 1-atm vertical gas mixing furnace in which the temperature was monitored using an S-type thermocouple. Mixtures of H 2 and CO 2 were used to control oxygen fugacity ( f O 2 ), which was monitored using a SIRO2 C700+ solid electrolyte oxygen sensor. The samples were at dwell temperatures ranging from 1,200 to 1,500 °C for up to 19 h ( Supplementary Table 3 ), after which they were quenched into water. Petrography and major element analysis The products of the synthesis runs were mounted in epoxy resin, polished and characterized using the UH JEOL JXA-8500F field emission electron microprobe (EMP) operating at 20 kV accelerating voltage, 50 nA beam current and 1−5 micron beam sizes. Counting times on both peak (and background) were 90 s (and 45 s) for Mg, Cr and Si, 30 s (and 15 s) for Ni and Mn, and 20 s (and 10 s) for Fe. Minerals with known chemical compositions were used as standards. The compositions of the olivine samples are described using their fayalite numbers. Liquidus olivine grains (Fa 31–99 ) obtained from partial melts are typically >100 μm in size and are compositionally uniform; they contain ∼ 0.7±0.1 wt% MnO and ∼ 0.06±0.03 wt% Cr 2 O 3 . The mineralogy and petrography of EET 90161, Semarkona, MET 00452, MET 96503, Ngawi, MAC 88107 and A-881317 were studied in transmitted and reflected light with an optical microscope and in backscattered electrons with the UH EMP. Quantitative chemical analyses were performed with the UH JEOL JXA-8500F EMP operated at 15 kV accelerating voltage, 15–20 nA beam current, and ∼ 1 μm beam size using five wavelength spectrometers. Minerals with known chemical compositions were used as standards. Matrix effects were corrected using the ZAF correction method [49] . Oxygen-isotope systematics Oxygen isotopic compositions of fayalite, magnetite and chondrule olivines were measured in situ by SIMS with the UH Cameca ims-1280 ion microprobe using two measurement protocols, depending on grain size. For grains >10 μm, an ∼ 0.8–1.2 nA Cs + primary ion beam was focused to a diameter of ∼ 5 μm and rastered over a ∼ 10 × 10 μm 2 area for pre-sputtering (120 s). After pre-sputtering, the raster size was reduced to ∼ 7 × 7 μm 2 for automated centring of the secondary ion beam followed by data collection. An energy window of ∼ 40 eV was used. A normal-incident electron flood gun was used for charge compensation with homogeneous electron density over a region ∼ 70 μm in diameter. Three oxygen isotopes ( 16 O − , 18 O − and 17 O − ) were measured in multicollection mode using multicollection Faraday cups and an axial electron multiplier (EM). The mass-resolving power for 17 O − and for 16 O − and 18 O − were set to ∼ 5,500 and ∼ 2,000, respectively. 16 OH − signal was monitored in every measured spot and was typically <10 6 counts per second, compared with typical 17 O − count rates of 2 × 10 5 counts per second. Contribution of 16 OH − onto 17 O − was corrected based on a peak/tail ratio. The correction was typically <0.1‰ ( ∼ 0.5‰ at most). Instrumental mass fractionation effects for fayalite, magnetite and chondrule olivine were corrected by analysing terrestrial fayalite, terrestrial magnetite and San Carlos olivine standards, respectively. The standards were analysed repeatedly before and after each run. Reported errors (2 σ ) include both the internal measurement precision and the external reproducibility ( ∼ 0.5–1.4‰ (2 σ ) in both δ 17 O and δ 18 O) of standard data obtained during a given session. For grains <10 μm in size, an ∼ 20–30 pA primary Cs + beam was focused to ∼ 1–2 μm. The three oxygen isotopes, 16 O − , 17 O − and 18 O − , were measured in multicollection mode using a multicollection Faraday cup, an axial EM and a multicollection EM, respectively. The internal and external reproducibility on the multiple analyses of the standards was ∼ 1–3‰ (2 σ ) for both δ 17 O and δ 18 O. Small grains (<10 μm) are generally very difficult to identify under the optical microscope of the ims-1280 ion microprobe. To measure such small grains, we used the UH JEOL-5900LV scanning electron microscope to mark the regions of interest. This is done by focusing the electron beam, centring the grain of interest in the field of view and then increasing the magnification so that the electron beam is effectively a spot on the centre of the grain. The electron beam removes adsorbed water on the carbon coating in such a way that it appears as a dark spot in 16 O − scanning ion image in the ion probe. Scanning 16 O − images are obtained by rastering the ∼ 20 pA ion beam over an ∼ 10 × 10 to 50 × 50 μm 2 square. After the mark is found using 16 O − scanning ion imaging, we centre the point of interest under the ion beam and then turn off the primary beam to prepare for measurement. The sputter rate of the rastered beam is sufficiently low that it does not completely remove the sample’s conductive coating during ion imaging. A conductive pathway therefore remains available for the duration of the oxygen-isotope measurements. After analysis, the location of each probe spot was re-imaged by electron microscopy to check for beam overlap between phases and to identify large cracks or impurities that may have affected the result. Mn–Cr isotope systematic Mn–Cr isotope data were collected in situ with the UH Cameca ims-1280 ion microprobe using two measurement protocols, depending on grain sizes. A 16 O − primary beam with a 100 pA current was focused into a spot ∼ 5 μm in diameter and used to collect data from terrestrial and meteoritic olivines (Fa 10–34 ), liquidus-phase synthetic olivines (Fa 31–99 ) and fayalites (Fa 95–100 ) from the carbonaceous chondrites A-881317 and MAC 88107. Owing to the small size of the fayalite grains (≤4–5 μm) in the OC EET 90161, their Mn–Cr isotope data were collected using a 16 O − primary beam with a 65–75 pA current focused into a spot ∼ 3 μm in diameter. The positive secondary ions were accelerated with 10 kV. A 50 eV energy window was used. Three chromium ions, 50 Cr + , 52 Cr + and 53 Cr + , were measured simultaneously using two multicollection EMs and an axial EM, respectively. Subsequently 55 Mn + was measured on the axial EM by peak-jumping. The mass-resolving power was set to ∼ 4,500 for 50 Cr + and 52 Cr + , and ∼ 6,000 for 53 Cr + and 55 Mn + . These settings were sufficient to separate the 50 Cr + , 52 Cr + , 53 Cr + and 55 Mn + ions from interfering species, including 52 CrH + . Isotopic data were typically collected over 125 cycles (EET 90161) and 100 cycles (A-881317 and MAC 88107). The chromium count rates collected during the first 25 cycles were often higher than during the remaining cycles, so the first 25 cycles were removed due to possible contamination. Corrections were made for both the EM background noises and dead times. Chromium-isotope and 55 Mn/ 52 Cr ratios were calculated from the total number of counts to suppress systematic bias caused by low count rates of chromium [50] , [51] . The measured 53 Cr/ 52 Cr ratios were corrected for instrumental mass fractionation determined by repeat analyses of synthetic fayalite (Fa 99 ; ref. 14 ), which was assumed to have a terrestrial 53 Cr/ 52 Cr ratio of 0.113459 (ref. 52 ). We could not do an internal mass fractionation correction because the interferences ( 50 V and 50 Ti) on 50 Cr were too large. The measured 55 Mn/ 52 Cr ratios were reduced using an RSF (defined here as ( 55 Mn + / 52 Cr + ) SIMS /( 55 Mn/ 52 Cr) EMPA ) determined on synthetic fayalite (Fa 99 ; ref. 14 ; Fig. 3 , Supplementary Table 4 and Supplementary Discussion ) that was measured daily and bracketed the unknown. The Fa 99 ( 55 Mn/ 52 Cr) EMPA ratio was calculated assuming 83.789 % of Cr is 52 Cr (ref. 53 ). As the ion yields changed with time, a time-averaged RSF was used. The measurement durations of the bracketing Fa 99 standards were matched to that of the unknown if (on the rare occasion) the meteoritic fayalite analysis was shortened (for example, owing to the base of the grain being breached). The reported uncertainties (2 σ ) in chromium-isotope ratio and 55 Mn/ 52 Cr ratio include both the internal precision of an individual analysis and the external reproducibility for standard measurements during a given analytical session. After analysis, the location of each probe spot was re-imaged by electron microscopy to check for beam overlap between phases and to identify large cracks or impurities that may have affected the result. Age anchors We used the U-isotope-corrected Pb–Pb absolute age of the CV CAIs (4,567.30±0.16 Ma; ref. 9 ) as the age of the Solar System. Owing to the presence of isotopically anomalous chromium, absence of primary minerals with Mn/Cr >>1 and evidence for a late-stage disturbance of 53 Mn– 53 Cr systematics in CV CAIs [20] , the initial 53 Mn/ 55 Mn ratio of the Solar System is not known. In this paper, relative 53 Mn– 53 Cr ages obtained in fayalites as well as those in calcites reported in literature [8] are anchored to the D’Orbigny angrite for which ( 53 Mn/ 55 Mn) 0 and U-corrected Pb–Pb absolute ages are known [21] , [22] . Angrites are a small but diverse group of igneous meteorites that are divided into two subgroups: coarse-grained plutonic and fine-grained quenched angrites (ref. 54 and references therein). The mineralogy, bulk chemical and isotopic compositions suggest that both subgroups originated on the same parent body. Crystallization of the quenched angrites predates that of the plutonic angrites by ∼ 7 Myr (refs 55 , 56 ). The quenched angrites are useful as age anchors for multiple short-lived chronometers (ref. 56 ) as (1) having crystallized from a melt, they were isotopically homogenized at the time of their original formation; (2) they formed sufficiently early in the history of the Solar System to contain measurable excesses of the daughter products of several short-lived radionuclides; and (3) they crystallized and cooled rapidly at the time of their formation, effectively closing the isotope systems of long- and short-lived chronometers at the same time. Among the quenched angrites dated, we used D’Orbigny as an age anchor for calculating model ages for the following reasons: (1) it is relatively unmetamorphosed, and therefore preserves the chronological records largely undisturbed [57] ; (2) it has a precise U-isotope-corrected Pb–Pb absolute age (4,563.37±0.25 Ma; ref. 22 ); and (3) very well-defined 53 Mn– 53 Cr isochron (( 53 Mn/ 55 Mn) 0 ratio of (3.24±0.04) × 10 −6 ; ref. 21 ). Anchoring the fayalite data to other plutonic anchors ( Supplementary Fig. 1 ) could result in a 1.4 Myr age difference, as discussed in the Supplementary Methods . The calculated 53 Mn– 53 Cr ages of fayalite were subsequently compared with the U-corrected Pb–Pb absolute age (4,567.30±0.16 Ma) of the CV CAIs [9] . We recalculated the previously reported model ages of secondary calcites in CM carbonaceous chondrites [8] relative to the D’Orbigny angrite anchor ( Supplementary Table 5 and Supplementary Fig. 2 ). Thermal modelling of chondrite parent bodies To model the thermal evolution of the L, CV and CO chondrite-like bodies consistent with the peak metamorphic temperatures, the temperature range of fayalite formation and the inferred 53 Mn– 53 Cr ages of fayalite crystallization, we considered spherically symmetric, instantaneously accreting bodies that were heated by decay of 26 Al only. A heat-conduction equation, where ρ is density, c is specific heat, T is temperature, t is time, r is radius from the centre, K is thermal conductivity, A is initial radiogenic heat generation rate per unit volume and λ is the decay constant of 26 Al, is solved numerically using a finite difference method and an explicit integral method [58] . We assumed that (1) 26 Al was the only heat source of a chondrite parent body, and was uniformly distributed in the protoplanetary disk with the canonical 26 Al/ 27 Al ratio of 5.25 × 10 −5 ; (2) some regions of these parent bodies reached 100−200 °C (temperature range of fayalite formation [28] ) at the time of fayalite formation; and (3) that these regions avoided subsequent heating above 300 °C (to preclude Fe–Mg diffusion in secondary fayalite). Supplementary Table 6 (part 1) defines parameters specific to the parent bodies from which the L, CV and CO chondrites were derived, such as the fayalite formation ages ( Figs 4 and 5 ) and peak metamorphic temperatures experienced by these parent bodies [23] , [31] , [32] . We note that using an initial 26 Al/ 27 Al ratio of 5.25 × 10 −5 , rather than 5 × 10 −5 , corresponds to 0.05 Myr, which is well within the uncertainty of our isotope measurements (0.4−1.8 Myr). The initial parameters (assumed to be constant) of the L, CV and CO chondrite parent bodies are detailed in Supplementary Table 6 (part 2; refs 28 , 59 ). In addition, we used the physical properties (thermal conductivity, specific heat and density) for ice, water [60] , [61] and rock [62] , [63] , detailed in Supplementary Table 6 (part 3). The latent heat of ice melting has been included, and we numerically calculated the effect of ice melting on the thermal evolution. Hydration reactions were not included, as the primary goal is to determine whether or not the parent bodies could reach the formation temperature range of fayalite. The thermal model also does not include the potential influence of an overlying regolith to reduce the thermal diffusivity. Two previous estimates of 26 Al heating of meteorite parent bodies [64] , [65] reported much higher temperatures than those calculated here, most likely owing to the differences in the assumed physical properties such as the thermal diffusivity (previous studies assumed values of <0.01) and the water/rock ratio (assumed to be zero in the previous studies). We note that increasing the water/rock ratio not only increases the amount of energy required to heat the parent body to a given temperature (ice has a higher heat capacity than rock) but also reduces the amount of 26 Al (per unit mass) available to produce heat as water does not contain any 26 Al. Parent bodies with radii of 20, 30, 40 and/or 50 km were modelled for the L, CV and CO chondrite parent bodies ( Fig. 6 ). The size of the bodies selected may also represent larger bodies as the maximum temperature reached by a parent body larger than 30 km in radius is largely independent of its size, and there is little difference in the accretion times of the larger bodies ( Fig. 6a,b ). How to cite this article: Doyle, P. M. et al. Early aqueous activity on the ordinary and carbonaceous chondrite parent bodies recorded by fayalite. Nat. Commun. 6:7444 doi: 10.1038/ncomms8444 (2015).